Generation of three-dimensional retinal tissue with functional photoreceptors from human iPSCs Many forms of blindness result from the dysfunction or loss of retinal photoreceptors. Induced pluripotent stem cells (iPSCs) hold great potential for the modelling of these diseases or as potential therapeutic agents. However, to fulfill this promise, a remaining challenge is to induce human iPSC to recreate in vitro key structural and functional features of the native retina, in particular the presence of photoreceptors with outer-segment discs and light sensitivity. Here we report that hiPSC can, in a highly autonomous manner, recapitulate spatiotemporally each of the main steps of retinal development observed in vivo and form three-dimensional retinal cups that contain all major retinal cell types arranged in their proper layers. Moreover, the photoreceptors in our hiPSC-derived retinal tissue achieve advanced maturation, showing the beginning of outer-segment disc formation and photosensitivity. This success brings us one step closer to the anticipated use of hiPSC for disease modelling and open possibilities for future therapies. Many retinal degenerative diseases are characterized by the dysfunction and death of photoreceptor cells, leading to vision loss and eventually total blindness [1] , [2] , [3] . Despite decades of research, there is currently no cure for these diseases. The establishment of human induced pluripotent stem cell (hiPSC) technology generated considerable excitement due to its potential for developing in vitro biological models and, eventually, therapeutic treatments for such diseases [4] , [5] , [6] , [7] , [8] , [9] . However, it is still unclear to what extent hiPSC may be capable of recapitulating in vitro the cellular and molecular features of the native retina, especially regarding photoreceptor differentiation and functional maturation. Several studies have shown that under specifically defined culture conditions, embryonic stem (ES) and induced pluripotent stem (iPS) cells can be induced to differentiate along a retinal lineage, including differentiation into photoreceptors [10] , [11] , [12] , [13] , [14] , [15] , [16] , [17] , [18] , [19] . Moreover, it has recently been shown that mouse and human ES cells can develop into a three-dimentional (3D) optic cup in culture that remarkably resembles the embryonic vertebrate eye [20] , [21] . Notwithstanding, the structural and molecular characteristics of advanced photoreceptor differentiation, including the formation of outer-segment discs—an essential structural feature for photoreceptor function—have yet to occur in vitro [6] , [7] , [8] , [9] . Perhaps as a consequence, no photoreceptor–light response has been observed in such cultures either. Finally, it remains to be determined whether iPSC can recreate the 3D histo-architecture of the neural retina (NR) in vitro beyond a rudimentary stratification [22] . Retinal cell differentiation in vivo takes place through sequential cell-fate specification steps, within a very dynamic and complex microenvironment involving highly coordinated cell–cell interactions through direct contact or diffusible signals [23] , [24] . Accordingly, in most published studies, differentiation of ES or iPS cells into retinal cells in vitro required an elaborate regime of exogenous factors [10] , [11] , [12] , [13] , [15] , [16] , [18] , [20] , [21] , [25] , [26] , [27] . Some studies, however, suggest that human ES and iPS cells have a certain propensity to differentiate into a retinal lineage [14] , [19] , [22] , [28] , [29] . Here we have succeeded in inducing human iPSC to recapitulate the main steps of retinal development and to form fully laminated 3D retinal tissue by exploiting the intrinsic cues of the system to guide differentiation ( Supplementary Fig. 1 ). Moreover, the photoreceptors in our preparations begin to develop outer-segment discs and reach the stage of photosensitivity. This highly autonomous system provides a powerful platform for developmental, functional and translational studies. Self-organized eye field domains Eye development in the embryo’s neural plate begins with the formation of the eye field (EF), a centrally organized domain consisting of a subpopulation of anterior neuroepithelial cells that have become further specified into retinal progenitors [23] , [30] ( Supplementary Fig. 1a ). The EF is characterized by the expression of a group of transcription factors that includes PAX6, RX, LHX2, SIX3 and SIX6, while the surrounding anterior neuroepithelial cells express PAX6 and SOX1 (refs 30 , 31 , 32 , 33 ). In parallel to the native events, our hiPSC-derived aggregates, after 8 days of differentiation (D8) in a chemically defined neural differentiation medium [14] , [22] , [29] and attached on Matrigel-coated culture dishes (see Methods for details), acquired an anterior neuroepithelial fate expressing PAX6 and SOX1 ( Fig. 1a–c ). Soon after, retinal progenitor cells expressing LHX2 appeared in the central region of the differentiating aggregates, concomitantly with a downregulation of SOX1 expression ( Fig. 1d ). By D12, EF-like domains with their characteristic flat, tightly packed appearance could be observed, surrounded by anterior neuroepithelial cells ( Fig. 1e,f ). Retinal progenitor cells within the EF domains lacked expression of SOX1 ( Fig. 1f ) and co-expressed the EF transcription factors PAX6, LHX2 and RX ( Fig. 1g,h ). The surrounding anterior neuroepithelial cells expressed SOX1 and PAX6 but were negative for LHX2 or RX, and typically formed rosettes ( Supplementary Fig. 2i–l ), which, although not found in the native situation, are characteristic of these cells in culture [14] , [34] . 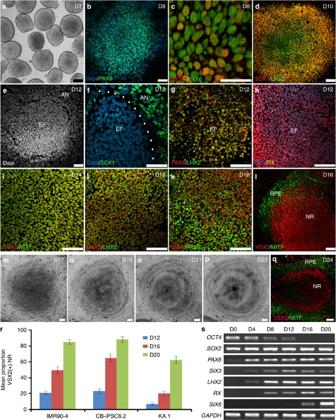Figure 1: hiPSC-derived retinal progenitors self-organized into EF-like domains and subsequently differentiated into NR and RPE. hiPSC-derived, free-floating aggregates (a) seeded in Matrigel-coated dishes acquired an anterior neuroepithelial (AN) fate characterized by SOX1/PAX6 expression (b,c); subsequently, retinal progenitors (LHX2-positive) first appeared in the centre of the aggregates (d). By D12, well-defined EF domains (e,f) expressing PAX6, LHX2 and RX (g,h) could be observed surrounded by AN cells (f). As differentiation progressed, cells within the EF domains co-expressed VSX2 and MITF (i), and afterwards differentiated into a central VSX2/LHX2/PAX6-positive NR domain (j–l) and a peripheral RPE domain expressing MITF but not VSX2 (l). (m–q) The NR domain progressively acquired an optic-cup-like shape. (r) Efficiency of NR domain formation among three hiPSC lines (mean±s.d., three experiments/time point/cell line). (s) Reverse transcription–PCR analysis showing progressive acquisition of retinal fate. Scale bars, 100 μm (aandm–p); 50 μm (b–landq). Figure 1: hiPSC-derived retinal progenitors self-organized into EF-like domains and subsequently differentiated into NR and RPE. hiPSC-derived, free-floating aggregates ( a ) seeded in Matrigel-coated dishes acquired an anterior neuroepithelial (AN) fate characterized by SOX1/PAX6 expression ( b , c ); subsequently, retinal progenitors (LHX2-positive) first appeared in the centre of the aggregates ( d ). By D12, well-defined EF domains ( e , f ) expressing PAX6, LHX2 and RX ( g , h ) could be observed surrounded by AN cells ( f ). As differentiation progressed, cells within the EF domains co-expressed VSX2 and MITF ( i ), and afterwards differentiated into a central VSX2/LHX2/PAX6-positive NR domain ( j – l ) and a peripheral RPE domain expressing MITF but not VSX2 ( l ). ( m – q ) The NR domain progressively acquired an optic-cup-like shape. ( r ) Efficiency of NR domain formation among three hiPSC lines (mean±s.d., three experiments/time point/cell line). ( s ) Reverse transcription–PCR analysis showing progressive acquisition of retinal fate. Scale bars, 100 μm ( a and m – p ); 50 μm ( b – l and q ). Full size image The reverse transcription–PCR analyses in Fig. 1s summarize the temporal sequence of events in our system, showing the gradual loss of pluripotency (downregulation of OCT4), the acquisition of neural fate (sustained SOX2 expression and appearance of PAX6) and the progressive differentiation into retinal progenitors. Interestingly, the chronology of expression of the EF transcription factors mimicked the in vivo situation, with initial expression of PAX6 and SIX3, followed by LHX2 and RX, and eventually SIX6 (refs 30 , 31 ). Thus, without the need of a regime of exogenous factors, hiPSC were able to differentiate into retinal progenitors that self-organized into EF-like domains surrounded by anterior neuroepithelial-like cells, presenting a cellular organization closely resembling the embryonic anterior neural plate where the EF forms in vivo . Self-driven differentiation into NR and RPE The EF in vivo gives rise to the left and right optic vesicles, with their respective retinal progenitors eventually forming the future NR and retinal pigment epithelium (RPE) ( Supplementary Fig. 1a ). Cell-fate specification into either NR or RPE is regulated critically by two transcription factors, VSX2 and MITF, which initially are co-expressed in the bipotent progenitor cells but subsequently become restricted to the NR and RPE, respectively [23] , [35] , [36] . Again, as in the native situation, the cells within the EF-like domains in our cultures followed the same differentiation sequence; namely, these cells initially expressed both VSX2 and MITF ( Fig. 1i ), but subsequently segregated into a central NR-like domain expressing PAX6, LHX2, RX and VSX2 ( Fig. 1j–l and Supplementary Fig. 2a–d ), and a peripheral RPE-like domain expressing MITF and PAX6 ( Fig. 1l and Supplementary Fig. 1e ). Between D17 and D25 in culture, these NR and RPE domains transitioned to an optic-cup-like structure, with the NR progressively acquiring a horseshoe-dome shape reminiscent of the inner wall of the optic cup, surrounded by the RPE ( Fig. 1m–q and Supplementary Figs 1f and 2e–h ). Similar results were obtained from three different hiPSC lines (IMR90-4 (ref. 37 ), CB-iPSC6.2 (ref. 38 ), KA.1 (ref. 39 ); Supplementary Table 1 ) with the efficiency of NR domain formation in D20 being 85.0±3.0%, 88.3±3.5% and 62.3±4.6%, respectively ( Fig. 1r ). Thus, in our cultures, retinal progenitors in the EF domains underwent spontaneous differentiation into NR and RPE efficiently and reproducibly, closely mimicking their in vivo topological organization. Formation of 3D retinal cups and self-lamination The optic-cup-like shape of the NR domains in our cultures made them easily identifiable and amenable to individual mechanical detachment and collection for further culture in suspension ( Fig. 2a , Supplementary Fig. 3 and Methods for details). The NR domains, collected on D21–D28, had a high enrichment of NR progenitors (71.0±7.3% VSX2-positive cells versus 19.0±7.2% MITF-positive cells, mean±s.d. ; Fig. 2b ) and, when cultured in suspension, formed 3D retinal cups (RCs) with an efficiency ranging from 50 to 70% (3 independent experiments with over 100 NR domains/experiment). The RC consisted of a thick, transparent NR that was continuous with the adjacent RPE, which appeared bundled at the tip of the RC and became gradually pigmented ( Fig. 2c,d ). From the time of NR domain collection to D35 (Week 5, or W5), the NR presented molecular and histological features resembling the actual features of the human embryonic retina at the same age [40] , including a polarized, pseudostratified epithelium with proliferating cells undergoing interkinetic nuclear migration and expressing the appropriate transcription factors ( Fig. 2e–k and Supplementary Movie 1 ). During W5–W7, the NR cells spontaneously began to differentiate, following the characteristic centre-to-periphery wave of neurogenesis and migrating to their corresponding retinal layers ( Fig. 3 ). 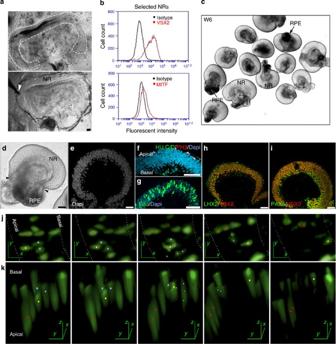Figure 2: Formation of 3D RCs. (a) One NR domain (top panel) is being detached with a tungsten needle (arrowhead in bottom panel). (b) Fluorescence-activated cell sorting analysis of collected NR domains showed enrichment in NR progenitors (VSX2-positive) compared with RPE progenitors (MITF-positive). (c) Detached NR domains cultured in suspension formed 3D RCs, composed of an NR epithelium and RPE (arrow). (d) Higher magnification of a typical 3D RC with an NR epithelium continuous with the adjacent RPE bundled at the tip (arrowheads). (e,f) The pseudostratified neural epithelium within the RC showed the typical polarity, with mitosis (Phospho-Histone H3 (PH3)-positive) occurring at the apical side and postmitotic neuronal precursors (HU C/D-positive) accumulating at the basal side. (g–i) NR cells proliferated actively (EdU-positive,g) and co-expressed transcription factors characteristic of neural retina progenitor cells (h,i). (j–k) Retinal progenitors within the NR epithelium underwent interkinetic nuclear migration. (j) Time-lapse imaging of retinal progenitors expressing nuclear green fluorescent protein (GFP). (k) Three-dimensional volume rendering of the cells shown in (j); red dot: cell undergoing mitosis; yellow dot: cell nucleus migrating from the apical to the basal side of the neuroepithelium; blue dots: cells undergoing apoptosis. Scale bars, 100 μm (aandc); 50 μm (d–i). Figure 2: Formation of 3D RCs. ( a ) One NR domain (top panel) is being detached with a tungsten needle (arrowhead in bottom panel). ( b ) Fluorescence-activated cell sorting analysis of collected NR domains showed enrichment in NR progenitors (VSX2-positive) compared with RPE progenitors (MITF-positive). ( c ) Detached NR domains cultured in suspension formed 3D RCs, composed of an NR epithelium and RPE (arrow). ( d ) Higher magnification of a typical 3D RC with an NR epithelium continuous with the adjacent RPE bundled at the tip (arrowheads). ( e , f ) The pseudostratified neural epithelium within the RC showed the typical polarity, with mitosis (Phospho-Histone H3 (PH3)-positive) occurring at the apical side and postmitotic neuronal precursors (HU C/D-positive) accumulating at the basal side. ( g – i ) NR cells proliferated actively (EdU-positive, g ) and co-expressed transcription factors characteristic of neural retina progenitor cells ( h , i ). ( j – k ) Retinal progenitors within the NR epithelium underwent interkinetic nuclear migration. ( j ) Time-lapse imaging of retinal progenitors expressing nuclear green fluorescent protein (GFP). ( k ) Three-dimensional volume rendering of the cells shown in ( j ); red dot: cell undergoing mitosis; yellow dot: cell nucleus migrating from the apical to the basal side of the neuroepithelium; blue dots: cells undergoing apoptosis. Scale bars, 100 μm ( a and c ); 50 μm ( d – i ). 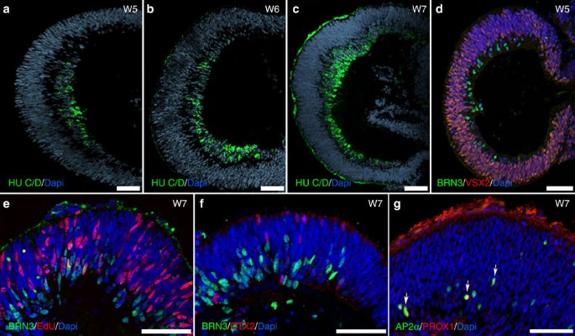Figure 3: Retinal progenitors within hiPSC-derived RCs underwent spontaneous differentiation. Retinal progenitors differentiated following the typical central-to-peripheral pattern (a–c) and acquired early-born cell fates, beginning with generation of ganglion cells (BRN3-positive/EdU-negative,d–f), followed by photoreceptors (OTX2-positive,f), amacrine cells (AP2α-positive,g) and horizontal cells (AP2α/PROX1-positive, arrows ing). Scale bars, 50μm. Full size image Figure 3: Retinal progenitors within hiPSC-derived RCs underwent spontaneous differentiation. Retinal progenitors differentiated following the typical central-to-peripheral pattern ( a – c ) and acquired early-born cell fates, beginning with generation of ganglion cells (BRN3-positive/EdU-negative, d – f ), followed by photoreceptors (OTX2-positive, f ), amacrine cells (AP2α-positive, g ) and horizontal cells (AP2α/PROX1-positive, arrows in g ). Scale bars, 50μm. Full size image Recapitulation of in vivo NR differentiation To promote cell survival beyond W7, the culture medium was supplemented with fetal bovine serum, taurine and retinoic acid (RA) until W17, at which time further slight modifications (less RA and replacement of the neurobasal supplement B27 by N2) were made to induce photoreceptor maturation (see Methods for details). These conditions allowed the RCs to maintain their shape and steady growth (with the longest axis increasing from 0.4±0.1 mm on D45 to 0.7±0.1 mm on D90, mean±s.d.) ( Fig. 4a–e ) and to develop distinguishable layers containing all major retinal cell types, including Müller cells ( Fig. 4f–j ). Ganglion cells first appeared in W5 ( Fig. 3d ) and over time increased in number and migrated towards the emerging ganglion cell layer ( Fig. 5a–c, e–g ), which became well established by W12–W13 ( Fig. 5d ), sometimes including a developing nerve-fibre-like layer ( Fig. 5h ). Photoreceptors (expressing OTX2) appeared during W7 and, over the subsequent weeks, populated the developing outer nuclear layer (ONL; where photoreceptor cell bodies are situated in the mature retina) and expressed recoverin, a well-known phototransduction protein ( Fig. 5a–c,e–g ). Amacrine cells (expressing AP2α) and horizontal cells (expressing PROX1) also appeared during W7 ( Fig. 5i ). As time progressed, amacrine and horizontal cells became numerous and began to segregate to their corresponding layers ( Fig. 5j–l ). By W21, the RCs presented a well-organized outer nuclear layer, adjoining a developing outer plexiform layer expressing the synaptic vesicle protein, SV2 ( Fig. 5m,n ). Rod opsin was also detectable in the distal part of photoreceptor cells ( Fig. 5o ). Finally, a developing bipolar cell layer containing postmitotic, VSX2-expressing bipolar cells appeared after W22 ( Fig. 5p ). This spatiotemporal pattern of differentiation closely mimics that of the vertebrate retina [41] , [42] and was observed in all of the RCs examined (~ 60) derived from the three different hiPSC lines used ( Fig. 5q and Supplementary Fig. 4 ). 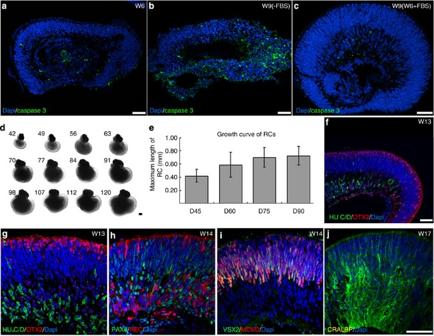Figure 4: Long-term suspension culture of hiPSC-derived RCs. (a–c) After W7, RCs progressively lost their histological organization due to increasing cell death (caspase 3-positive,a,b), which was avoidable by supplementation with fetal bovine serum, taurine and RA from the beginning of W7 onward (c). (d,e) Under these conditions, RCs maintained their shape, cellular organization and steady growth during long-term culture (bars: mean±s.d.; 15–20 RCs per time point). (f–i) By W13–W14, RCs showed distinguishable layers containing the precursors of most of the major neuronal cell types, including ganglion, amacrine and horizontal cells (HU C/D- and PAX6-positive), and photoreceptors (OTX2- and recoverin-positive); as in the developing human retina, cells expressing OTX2 and recoverin were observed in the developing outer nuclear layer as well as in the inner side of the retinal epithelium69,70. A conspicuous neuroblastic layer containing mitotic retinal progenitors (VSX2/MCM2-positive) was still present by W14 (i). (j) Müller cells expressing CRALBP were first seen by W17. Scale bars, 200 μm (d); 50 μm (a–candf–j). Figure 4: Long-term suspension culture of hiPSC-derived RCs. ( a – c ) After W7, RCs progressively lost their histological organization due to increasing cell death (caspase 3-positive, a , b ), which was avoidable by supplementation with fetal bovine serum, taurine and RA from the beginning of W7 onward ( c ). ( d , e ) Under these conditions, RCs maintained their shape, cellular organization and steady growth during long-term culture (bars: mean±s.d. ; 15–20 RCs per time point). ( f – i ) By W13–W14, RCs showed distinguishable layers containing the precursors of most of the major neuronal cell types, including ganglion, amacrine and horizontal cells (HU C/D- and PAX6-positive), and photoreceptors (OTX2- and recoverin-positive); as in the developing human retina, cells expressing OTX2 and recoverin were observed in the developing outer nuclear layer as well as in the inner side of the retinal epithelium [69] , [70] . A conspicuous neuroblastic layer containing mitotic retinal progenitors (VSX2/MCM2-positive) was still present by W14 ( i ). ( j ) Müller cells expressing CRALBP were first seen by W17. Scale bars, 200 μm ( d ); 50 μm ( a – c and f – j ). 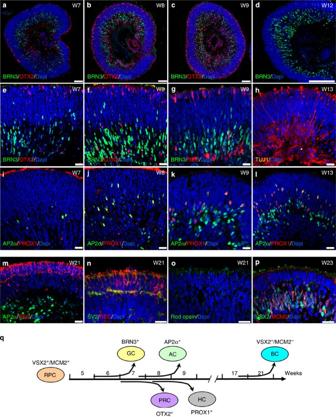Figure 5: hiPSC-derived NR progenitors within the 3D RCs recapitulated the spatiotemporal pattern of NR differentiationin vivo. (a–l) Cells within the RCs differentiated and migrated to their corresponding layers, with ganglion cells (GCs; BRN3-positive, (a–g); TUJ1-positive,hwhere * indicates a developing nerve-fibre-like layer) appearing first, followed by photoreceptor cells (PRC; OTX2/recoverin-positive,a–c,e–g), amacrine cells (AC; AP2α-positive,i–l) and horizontal cells (HC; PROX1-positive,i–l). (m–p) By W21–W23, RCs presented a well-established outer nuclear layer (REC-positive,m,n) delineated by a developing outer plexiform layer (SV2-positive,n) and containing rod opsin-positive photoreceptors (o) and a developing bipolar cell layer containing bipolar cells (BC; VSX2-positive/MCM2-negative,p) intermingled with the remaining retinal progenitor cells (RPC; VSX2-positive/MCM2-positive,p). (q) Timeline of retinogenesis in hiPSC-derived 3D RCs. Scale bars, 100 μm (a–d); 20 μm (e–p). Full size image Figure 5: hiPSC-derived NR progenitors within the 3D RCs recapitulated the spatiotemporal pattern of NR differentiation in vivo . ( a – l ) Cells within the RCs differentiated and migrated to their corresponding layers, with ganglion cells (GCs; BRN3-positive, ( a – g ); TUJ1-positive, h where * indicates a developing nerve-fibre-like layer) appearing first, followed by photoreceptor cells (PRC; OTX2/recoverin-positive, a – c , e – g ), amacrine cells (AC; AP2α-positive, i – l ) and horizontal cells (HC; PROX1-positive, i – l ). ( m – p ) By W21–W23, RCs presented a well-established outer nuclear layer (REC-positive, m , n ) delineated by a developing outer plexiform layer (SV2-positive, n ) and containing rod opsin-positive photoreceptors ( o ) and a developing bipolar cell layer containing bipolar cells (BC; VSX2-positive/MCM2-negative, p ) intermingled with the remaining retinal progenitor cells (RPC; VSX2-positive/MCM2-positive, p ). ( q ) Timeline of retinogenesis in hiPSC-derived 3D RCs. Scale bars, 100 μm ( a – d ); 20 μm ( e – p ). Full size image Rod-dominant ONL with highly differentiated rods and cones Although photoreceptors expressed detectable levels of rod opsin in the culture conditions described above, further developmental maturation, including the formation of outer-segment discs, did not appear to progress. In addition, expression of L/M- and S-cone opsins was not apparent. As RA has been shown to influence photoreceptor differentiation in a time- and concentration-dependent manner [43] , we reasoned that prolonged exposure to a relatively high retinoic acid concentration (1 μM RA in W7–W17) might hamper photoreceptor maturation. Accordingly, we tested two shorter time windows of retinoic acid exposure (W7–W14 and W10–W14, both with 1 μM RA) in CB-iPSC6.2-derived RCs ( Fig. 6 ). The W10–W14 condition induced, already at W17, the appearance of dispersed cells showing high rod-opsin expression not only in the distal part of the immature photoreceptors but also in their cell bodies, as seen in native development [44] (observed in ~33% of the RCs, n =12; Figs 6a and 7a–c ). Moreover, we also began to observe S-opsin expression in some photoreceptors not expressing rod opsin ( Fig. 7d ). By W21, 90% of the hiPSC-derived RCs ( n =20) showed a significant increase in the number of photoreceptors expressing rod opsin, organized in patches throughout the outer nuclear layer or even encompassing the full extent of this layer ( Fig. 7e ). Photoreceptors expressing L/M- or S-opsins were also observed ( Fig. 7f–i ). The morphologies of the rods and cones and the localization of their cell bodies, with cones at the outer edge and rods toward the inner edge of the outer nuclear layer, resembled remarkably the native situation [44] ( Fig. 7g–i and Supplementary Movie 2 ). The photoreceptors showed bud-like structures at their distal tip reminiscent of the short nascent outer segments at comparable developmental stages in the human retina [44] , [45] , [46] ( Fig. 7g–i and Supplementary Movie 2 ). Rarely, elongated structures resembling more advanced native outer segments were seen in W25 (arrow in Fig. 7j ). A similar pattern of photo-pigments expression was observed in RCs derived from the three cell lines tested upon W10–W14 RA treatment ( Fig. 6b–g ), albeit with different efficiencies as evaluated for rod opsin expression at W21 (90, 47 and 38% of cups from CB.iPS6.2 ( n =20), IMR90-4 ( n =22) and KA.1 ( n =8), respectively). 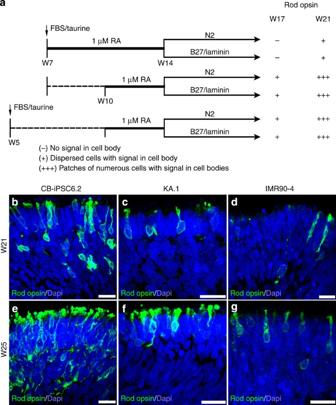Figure 6: Effect of RA on the differentiation of hiPSC-derived photoreceptors. (a) Two windows of exposure to 1 μM RA were tested in combination with slight modifications to the culture media in CB-iPSC6.2-derived RCs. RA treatment in W7–W14 led to low levels of rod opsin expression in the distal part of photoreceptor cells as observed in the original culture conditions, except for some RCs that showed few cells with rod opsin expression in the cell bodies at W21. In contrast, RCs treated during W10–W14 showed dispersed cells with strong rod opsin expression in their cell bodies already at W17, and forming large patches at W21. We did not observe significant differences associated with modifications of the culture media after RA treatment or presence of fetal bovine serum/Taurine from W5. Similar results were observed in three independent experiments, five RCs per treatment per time window. (b–g) When KA.1- and IMR90-4-derived RCs were subjected to RA treatment in W10–W14, induction of rod opsin expression was also observed, although less efficiently than in CB-iPSC6.2-derived RCs (3 independent experiments, 8–22 RCs per cell line). Scale bars, 20 μm. Figure 6: Effect of RA on the differentiation of hiPSC-derived photoreceptors. ( a ) Two windows of exposure to 1 μM RA were tested in combination with slight modifications to the culture media in CB-iPSC6.2-derived RCs. RA treatment in W7–W14 led to low levels of rod opsin expression in the distal part of photoreceptor cells as observed in the original culture conditions, except for some RCs that showed few cells with rod opsin expression in the cell bodies at W21. In contrast, RCs treated during W10–W14 showed dispersed cells with strong rod opsin expression in their cell bodies already at W17, and forming large patches at W21. We did not observe significant differences associated with modifications of the culture media after RA treatment or presence of fetal bovine serum/Taurine from W5. Similar results were observed in three independent experiments, five RCs per treatment per time window. ( b – g ) When KA.1- and IMR90-4-derived RCs were subjected to RA treatment in W10–W14, induction of rod opsin expression was also observed, although less efficiently than in CB-iPSC6.2-derived RCs (3 independent experiments, 8–22 RCs per cell line). Scale bars, 20 μm. 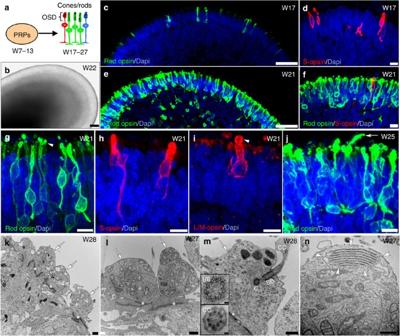Figure 7: hiPSC-derived rod and cone photoreceptors achieved an advanced level of differentiation including outer-segment disc formation. (a) During normal development photoreceptor precursors (PRPs) differentiate into rods, L/M- and S-cones (in green, red and blue colour, respectively). (b) A W22 CB-iPSC6.2-derived RC that has been exposed to 1-μM RA in W10–W14. (c–j) Under this condition, photoreceptors expressing high levels of rod opsin in the entire cell body were first observed by W17 (c), significantly increasing in number and forming large patches by W21 (e,f). S-opsin expression could be observed in some rod opsin-negative photoreceptors (d,f). High-magnification images of W21 RCs showing rods (g), S- (h) and L/M- (i) cones with a morphology and a topological organization similar to those of thein vivoretina44, including structures reminiscent of short, nascent outer segments (arrowheads). By W25, elongated structures resembling more developed outer segments were rarely observed (j, arrow). (k–n), Transmission electron microscopic analysis revealed the presence of an outer limiting membrane (*), inner segments (arrows), basal bodies (BB), connecting cilia (CC) and stacks of outer-segment discs (demarcated by arrowheads). BB and CC presented the photoreceptor-specific microtubule arrangement consisting of 9 × 3+0 and 9 × 2+0, respectively (inserts inm). C, centriole. Scale bars, 50 μm (b,c,e); 10 μm (d,fandg–j); 0.5 μm (k–n); 0.05 μm (minserts). Full size image Figure 7: hiPSC-derived rod and cone photoreceptors achieved an advanced level of differentiation including outer-segment disc formation. ( a ) During normal development photoreceptor precursors (PRPs) differentiate into rods, L/M- and S-cones (in green, red and blue colour, respectively). ( b ) A W22 CB-iPSC6.2-derived RC that has been exposed to 1-μM RA in W10–W14. ( c – j ) Under this condition, photoreceptors expressing high levels of rod opsin in the entire cell body were first observed by W17 ( c ), significantly increasing in number and forming large patches by W21 ( e , f ). S-opsin expression could be observed in some rod opsin-negative photoreceptors ( d , f ). High-magnification images of W21 RCs showing rods ( g ), S- ( h ) and L/M- ( i ) cones with a morphology and a topological organization similar to those of the in vivo retina [44] , including structures reminiscent of short, nascent outer segments (arrowheads). By W25, elongated structures resembling more developed outer segments were rarely observed ( j , arrow). ( k – n ), Transmission electron microscopic analysis revealed the presence of an outer limiting membrane (*), inner segments (arrows), basal bodies (BB), connecting cilia (CC) and stacks of outer-segment discs (demarcated by arrowheads). BB and CC presented the photoreceptor-specific microtubule arrangement consisting of 9 × 3+0 and 9 × 2+0, respectively (inserts in m ). C, centriole. Scale bars, 50 μm ( b , c , e ); 10 μm ( d , f and g – j ); 0.5 μm ( k – n ); 0.05 μm ( m inserts). Full size image Acquisition of functional photoreceptors Possibly one of the most challenging and still unresolved issues is whether photoreceptors derived from ES and/or iPS cells in vitro are capable of achieving functional maturation, that is, forming outer segments and responding to light [6] , [7] , [8] , [9] . We thus set out to evaluate these events in our system. During W27–W28, several ultrastructural features characteristics of advanced differentiation were revealed by electron microscopy, including an outer limiting membrane, inner segments with numerous mitochondria and basal bodies with connecting cilia having a photoreceptor-specific microtubule arrangement ( Fig. 7k–m ). Although at low frequency, some photoreceptors also showed intracellular membrane discs reminiscent of the outer-segment discs in native photoreceptors ( Fig. 7n and Supplementary Fig. 1j ; average of developing outer-segment disc stacks observed: 2 per 150 μm of ONL length; n =4 ultra-thin sections). All of these features were very similar to those observed in the developing human retina [47] , [48] . Perhaps more importantly, several key proteins involved in rod phototransduction were expressed in the photoreceptors of W25 hiPSC-derived RCs, including the α-subunit of rod transducin (G T1α ), the α- and β-subunits of the rod cGMP-phosphodiesterase (PDE6 αβ ), the rod cyclic-nucleotide-gated channel α-subunit and β-subunit, and retinal guanylate cyclase 1 ( Fig. 8a–i ). These proteins increased in expression over time in parallel to rod opsin, as in native human retina [44] ( Supplementary Fig. 5a–i ). 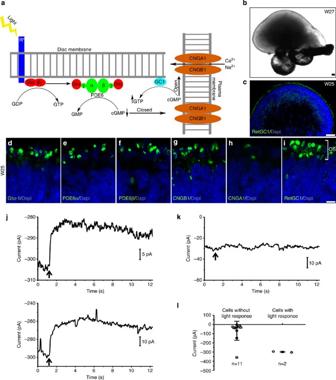Figure 8: hiPSC-derived photoreceptors expressed proteins of the phototransduction pathway and occasionally showed light responsein vitro. (a) Diagram of rod phototransduction pathwayin vivo. (b) Three-dimensional RCs still maintained their structural organization in W27. (c–i) Photoreceptors within the RCs showed expression of phototransduction proteins with the appropriate cellular distributions (OS: putative developing outer segments). (j–l) Perforated-patch electrophysiological recordings from CB-iPSC6.2-derived photoreceptors, showing the flash-triggered responses (single trial) from two light-sensitive cells (j), the lack of flash response from one light-insensitive cell (k) and collected data from 13 cells (l). Cells were voltage clamped at −50 mV. Inward current is negative. Flash (indicated by arrow) was 40 ms in duration and 2.46 × 105μW cm−2in intensity (white light from a mercury arc lamp). Inl, open circles indicate individual cells, solid circles indicate mean values and error bars indicate s.d. Scale bars, 50 μm (b,c); 5 μm (d–i). Figure 8: hiPSC-derived photoreceptors expressed proteins of the phototransduction pathway and occasionally showed light response in vitro . ( a ) Diagram of rod phototransduction pathway in vivo . ( b ) Three-dimensional RCs still maintained their structural organization in W27. ( c – i ) Photoreceptors within the RCs showed expression of phototransduction proteins with the appropriate cellular distributions (OS: putative developing outer segments). ( j – l ) Perforated-patch electrophysiological recordings from CB-iPSC6.2-derived photoreceptors, showing the flash-triggered responses (single trial) from two light-sensitive cells ( j ), the lack of flash response from one light-insensitive cell ( k ) and collected data from 13 cells ( l ). Cells were voltage clamped at −50 mV. Inward current is negative. Flash (indicated by arrow) was 40 ms in duration and 2.46 × 10 5 μW cm −2 in intensity (white light from a mercury arc lamp). In l , open circles indicate individual cells, solid circles indicate mean values and error bars indicate s.d. Scale bars, 50 μm ( b , c ); 5 μm ( d – i ). Full size image To determine whether the photoreceptors in our RCs had the ability to respond to light, we conducted perforated-patch recordings in the voltage-clamp mode from the putative rod cells in W25–W27 hiPSC-derived RCs. We found 2 out of 13 randomly chosen cells to respond to a light flash ( Fig. 8j ; an unresponsive cell is shown in Fig. 8k ). Considering that in these samples the outer segments were just beginning to appear (as inferred from the ultrastructural features described above), the infrequent encounter of light responsiveness is not too surprising. The light response consisted of an outward current (equivalent to the reduction of a steady inward current in darkness, similar to the situation in native rods) and the speed of the response’s rising phase also resembled that of the native response. The photosensitivities of the two responsive cells were much lower than those observed in adult-primate photoreceptors [49] , likely to be because the rod opsin level was still low and the downstream phototransduction steps were still maturing [50] , [51] , [52] . Repeated flashes failed to elicit further responses, perhaps because of functional depletion of the nascent phototransduction components. In darkness, a steady inward current was observed in practically all 13 cells recorded, and the 2 photoresponsive cells happened to have large inward currents ( Fig. 8l ) (see also ref. 30 for a cGMP-induced current in their preparations). The implication of the typically larger inward current of the photoresponsive cells is at present unclear because the current at this stage may have more than one component. Compared with the progressive maturation of photoreceptors, most ganglion cells and amacrine cells, on the other hand, gradually disappeared from the advanced cultures, presumably because they needed additional factors for their long-term survival. We have established a simple and efficient strategy for inducing hiPSC to differentiate almost autonomously into 3D retinal tissue in vitro , with spatial and temporal features that replicate the development of the human retina in vivo . Furthermore, the photoreceptors in our system are able to reach an advanced stage of maturation, up to at least the beginning of outer-segment formation and of photosensitivity. To our knowledge, this is the first demonstration that such a developmental step can be achieved in vitro . Differentiation of ES and iPS cells into retinal cells in vitro most commonly requires the use of extrinsic chemical factors to modulate specific signalling pathways, and to mimic the in vivo microenvironment where retinal cell specification normally occurs. In such protocols, the induction of retinal progenitor fate is achieved by adding combinations of bone morphogenetic protein, Wnt, Nodal and Notch pathway inhibitors (such as Noggin, Dkk1, LeftyA and DAPT), several growth factors (including insulin-like growth factor 1, basic fibroblast growth factor (FGF), activin, sonic hedgehog (SHH) and T3) and serum [10] , [11] , [12] , [13] , [15] , [16] , [26] , [27] . Further differentiation into photoreceptors has additionally required exposure to native retinal cells in co-culture systems or to several exogenous factors, including Noggin, Dkk1, DAPT, insulin-like growth factor 1, acidic FGF, basic FGF, T3, SHH, RA and taurine [10] , [11] , [12] , [13] , [15] , [16] , [26] , [27] . Similarly, the recent derivation of optic-cup-like structures from human ES cells required an elaborate differentiation strategy involving initial dissociation followed by re-aggregation of human ES cells and a rigorous regime of exogenous factors and long-term culture under high-oxygen conditions [21] . Conversely, Meyer et al . [14] reported the ability of select human ES and iPS cell lines to differentiate into retinal progenitor cells without the need of exogenous factors. These cells in turn were capable of forming optic vesicle-like structures with rudimentary lamination [22] , [29] . Building on these observations, here we succeeded in establishing a system in which without requiring extrinsic signalling modulators, human iPSCs differentiate into retinal progenitors and subsequently form 3D RCs capable of recreating the full histo-architecture of the native retina. Serum, taurine and RA are added at later times to promote cell survival, allowing spontaneous differentiation to proceed in a prolonged manner. Stem-cell-derived retinal progenitors in two-dimensional conditions have been shown to generate only certain retinal cell types, such as RPE, ganglion and photoreceptor cells, and they are most often found within mixed cell populations lacking tissue architectural features [10] , [11] , [12] , [13] , [15] , [16] , [26] . On the other hand, the human stem-cell-derived 3D retinal tissues reported to date showed relatively organized ganglion and outer nuclear layers with an intermediate layer mostly containing retinal precursors [21] , [22] . Sparse interneuron precursors representing horizontal and/or amacrine cells were also seen, but bipolar and Müller cells were lacking, as well as clearly defined amacrine, horizontal, bipolar and plexiform layers [21] , [22] . In contrast, human iPSC-derived retinal progenitors within our 3D RCs generated all major retinal cell types, including neurons (ganglion, amacrine, horizontal, bipolar, rod and the three types of cones) and Müller glial cells, all arranged in their proper layers. Taken together, our results suggest that under appropriate conditions, hiPSC have the potential to re-create a ‘retina-differentiation niche’ sufficient for inducing fully specified retinal progenitor cells capable of originating the entire repertoire of retinal cell types while recapitulating in time and space the development of the human retina. We speculate that physical microenvironmental cues (especially cell–cell and cell–extracellular matrix interactions [18] , [53] , [54] ) at the initial stages of hiPSC differentiation are key to the establishment of this retina-differentiation niche. Further evidence of the potential of hiPSC to re-enact retinal developmental processes in our system comes from the ability of hiPSC-derived photoreceptors to form outer-segment discs and elicit a light response, events that have not been achieved in vitro until our present study. The onset of outer-segment disc morphogenesis in the developing human retina occurs around fetal week 23–25, resulting in a small number of photoreceptors bearing bud-like outer-segment precursors [45] , [46] . The number of outer-segment precursors in vivo slowly increases over the following weeks and outer segment elongation does not start until about fetal week 32 (ref. 55 ). This is in agreement with the relatively infrequent observation of developing outer-segment discs in our samples at W27–W28. Assuming that the development of light-responsiveness parallels that of the outer segment, as previous studies have shown [50] , [51] , [56] , our infrequent observation of the light response is to be expected. There is no published information regarding the appearance of the light response in pre-term human fetus for comparison with our functional observation; electroretinographic recordings have been made only from human infants beginning at a few days postbirth [51] , [52] . Nonetheless, the studies in infants show that immature photoreceptors have a significantly lower sensitivity to light compared with those in the adult, associated to their lower concentrations of rhodopsin and other phototransduction proteins, and their shorter outer segments [51] , [52] , [57] . The advanced level of maturation of the hiPSC-derived photoreceptors in our cultures might result from the combined effects of the fairly autonomous 3D differentiation, the temporally extended culture and the timing/period of exposure to RA. A contribution from a cell-line-dependent effect, as observed in other studies [29] , [58] , cannot be ruled out, considering the differences in efficiency of rod opsin expression among the three cell lines tested. The importance of the native microenvironment on stem-cell-derived photoreceptor differentiation is supported by previous work using co-culture systems or subretinal transplantation [10] , [11] , [15] , [17] . In our system, the lack of extrinsic factors at the early stages of differentiation (which, while promoting a particular fate may also hinder other aspects of the developmental potential of the cells) and the 3D tissue organization achieved may contribute to creating a microenvironment very similar to that found within the native retina and to trigger the innate developmental programmes leading to photoreceptor functional differentiation. This is further supported by the time-dependent effect of RA on photoreceptor differentiation observed in our cultures, which correlates with a similar effect in the in vivo vertebrate retina [43] , [59] . Our culture conditions also permitted growth of the 3D RCs for a significantly longer time period compared with previous 3D systems [21] , [22] while preserving their histological features, thus allowing cells to reach a developmental stage comparable to that at which functional maturation of the photoreceptors begins in the human retina [45] , [46] , [55] . It is interesting that in our cultures a relatively advanced photoreceptor differentiation was achieved without physical contact with the RPE, as the RPE in our samples was bundled at the tip of the RC far away from the photoreceptors containing developing outer segments (we did not observe RPE, pigmented or non-pigmented, lining the apical surface of the NR at any time during differentiation, as evaluated by morphology, immunohistochemistry and transmission electron microscopy). Previous studies have indicated that RPE–photoreceptor cell contact and RPE-secreted factors are both important for photoreceptor differentiation and maturation [60] , [61] , [62] , [63] , [64] , [65] . Although the presence of diffusible RPE-derived factors in our cultures might have contributed to recreating a native-like environment propitious for photoreceptor differentiation, our observations suggest that physical contact with the RPE may not be required at least up to the beginning of their functional maturation. Finally, our system provides an in vitro model of human retina development where each of the main developmental stages can be easily identified by their morphology and independently manipulated. Furthermore, the success here with human iPSC opens up many exciting possibilities in establishing in vitro models for human eye diseases, including those associated with different aspects of photoreceptor functionality, and hopefully will also take potential therapeutic applications one step closer to reality. hiPSC culture Three hiPSC lines, IMR90-4 (ref. 37 ) (WiCell), CB-iPSC6.2 (ref. 38 ) and KA.1 (refs 39 , 66 ), were used in this study ( Supplementary Table 1 ). All cell lines were obtained with verified normal karyotype and were contamination free. hiPSCs were maintained on Matrigel (growth-factor-reduced; BD Biosciences)-coated plates with mTeSR1 medium (Stemcell Technologies) according to WiCell protocols. Cells were passaged every 5–7 days at ~80% confluence. Colonies containing clearly visible differentiated cells were marked and mechanically removed before passaging. The use of hiPSCs in this study conforms to The Johns Hopkins Institutional Stem Cell Research Oversight Committee. Early stages of retinal differentiation The procedure to induce early stages of retinal differentiation was based on a previously described protocol with major modifications [14] , [22] , [29] . Briefly, on day 0 (D0) of differentiation, hiPSCs were enzymatically detached by dispase treatment, dissociated into small clumps and cultured in suspension with mTeSR1 medium and 10 μM Blebbistatin (Sigma) to induce aggregate formation. Aggregates were gradually transitioned into neural-induction medium (NIM) containing DMEM/F12 (1:1), 1% N2 supplement (Invitrogen), 1 × minimum essential media-non essential amino acids (NEAAs), 2 μg ml −1 heparin (Sigma), by replacing the medium with a 3:1 ratio of mTeSR1/NIM on D1, 1:1 on D2 and 100% NIM on D3. On D7, aggregates (average size of 0.22±0.05 mm) were seeded onto Matrigel (growth-factor-reduced; BD Biosciences)-coated dishes containing NIM at an approximate density of 20 aggregates per cm 2 and switched to DMEM/F12 (3:1) supplemented with 2% B27 (without vitamin A, Invitrogen), 1 × NEAA and 1% antibiotic–antimycotic (Gibco) on D16. Thereafter, the medium was changed daily. Formation of 3D RCs On the fourth week of differentiation, horseshoe-shaped NR domains were manually detached with a sharpened Tungsten needle under inverted microscope, collected and cultured in suspension at 37 °C in a humidified 5% CO 2 incubator in DMEM/F12 (3:1) supplemented with 2% B27, 1 × NEAA, and 1% antibiotic–antimycotic, where they gradually formed 3D RCs. Thereafter, the medium was changed twice a week. For long-term suspension culture, the medium was supplemented with 10% fetal bovine serum (Gibco), 100 μM Taurine (Sigma) and 2 mM GlutaMAX (Invitrogen) beginning on D42, unless otherwise noted. RA treatment To promote photoreceptor maturation, suspension cultures of RCs were supplemented daily with 1 μM all-trans RA (Sigma) at various time windows: W7–W17, W7–W14 or W10–W14; subsequently, RA concentration was decreased to 0.5 μM. Immunohistochemistry Cells growing on adherent conditions were fixed in 4% paraformaldehyde (PFA; Sigma) for 15 min. RCs were fixed in 4% PFA for 30 min. A human eyeball from a 71-year-old person affected by age-related macular degeneration (Old Dominion Eye Foundation) was fixed in 4% PFA for 4 h. Tissue cryopreservation, sectioning and immunohistochemistry were performed as previously described [67] . Antibodies against the following proteins were used at the indicated dilutions: LHX2 (goat, 1:200, Santa Cruz, sc-19344), RX (rabbit, 1:500, Abcam, ab86210), SOX1 (goat, 1:1,000, R&D, AF3369), VSX2 (sheep, 1:500, Millipore, AB9016), OTX2 (rabbit, 1:500, Millipore, AB9566), recoverin (REC, rabbit, 1:500, Millipore, AB5585), Caspase 3 (rabbit, 1:500, Cell Signaling, asp175), HU C/D (mouse, 1:200, Molecular Probes, MP21271), BRN3 (goat, 1:1,000, Santa Cruz, sc-6026X), TUJ1(rabbit, 1:2,000, Covance, MRB-435P), MITF (mouse, 1:50, NeoMarkers, MS-771-P1), PROX1 (rabbit, 1:2,000, Millipore, AB5475), CRALBP (mouse, 1:500, Abcam, ab15051), rod opsin (mouse, 1:100, gift from Dr David Hicks), L/M-opsin (rabbit, 1:50,000, gift from Dr Jeremy Nathans), S-opsin (rabbit, 1:50,000, gift from Dr Jeremy Nathans), phosphodiesterase 6- α (rabbit, 1:1,000, Abcam, ab5659) and -β (rabbit, 1:2,000, Thermo Scientific, PA1-722), human retinal guanylate cyclase 1 (rabbit, 1:4,000, gift from Dr Alexander M. Dizhoor), G T1α (rabbit, 1: 2,000, Santa Cruz, sc-389), rod cyclic-nucleotide-gated channel α-subunit (mouse,1:10, a gift from Dr Robert S. Molday) and β-subunit (mouse, 1:10, a gift from Dr Robert S. Molday). Antibodies from the Developmental Studies Hybridoma Bank, developed under the auspices of the Eunice Kennedy Shriver National Institute of Child Health and Human Development and maintained by the Department of Biology, University of Iowa, were: PAX6 (mouse, 1:50), AP2α (3B5a, mouse, 1:35) and SV2 (mouse, 1:1,000). Secondary antibodies used included the corresponding species-specific Alexa Fluor-488-, -546- and -647-conjugated antibodies (1:500, Molecular Probes). DAPI (4',6-diamidino-2-phenylindole) was used for nuclear counterstaining (Molecular Probes). Fluorescence images were acquired with an LSM 510 confocal microscope (Zeiss). Detection of proliferating cells Click-iT EdU imaging kit (Invitrogen, C10337) was used according to the manufacturer’s protocol to visualize cells undergoing S-phase during the time window under study. Three-dimensional RCs were incubated with 50 μg of EdU diluted in PBS for 1 or 20 h, then collected and processed for microscopic imaging. An antibody against the DNA replication licensing factor MCM2 (rabbit, 1:1,000, Abcam, ab4461) was used to identify proliferating retinal progenitors, whereas an antibody against Phospho-Histone H3 (rabbit, 1: 250, Cell Signaling, #9701L) was used to identify cells in M-phase by immunohistochemistry as described above. Reverse transcription–PCR Total RNA isolation was done in triplicate with RNAeasy mini kit (Qiagen) and followed by DNase I treatment (Qiagen) to remove potential DNA contamination. RNA quality was evaluated using a NanoDrop1000 spectrophotometer (Thermo Scientific). Reverse transcription was performed using the SuperScript III reverse transcription–PCR kit (Invitrogen). Samples without reverse transcriptase were used as negative controls. PCR was performed with Taq DNA polymerase (Invitrogen) on a PTC-200 Thermal Cycler (Bio-Rad). Cycles (30–40 depending on primer pair) were run at 95 °C denaturation for 20 s, at 60 °C annealing for 20 s and at 72 °C extension for 30 s. Subsequent PCR products were run on 2% agarose gels. Primers used were as follows: OCT4 forward 5′-CGAGCAATTTGCCAAGCTCCTGAA-3′, reverse 5′-TCGGGCACTGCAGGAACAAATTC-3′; SOX2 forward 5′-CCCCCGGCGGCAATAGCA-3′, reverse 5′-TCGGCGCCGGGGAGATACAT-3′; PAX6 forward 5′-CGGAGTGAATCA GCTCGGTG-3′, reverse 5′-CCGCTTATACTGGGCTATTTTGC-3′; SIX3 forward 5′-CCGGAAGAGTTGTCCATGTT-3′, reverse 5′-CGACTCGTGTTTGTTGATGG-3′; LHX2 forward 5′-CAAGATCTCGGACCGCTACT-3′, reverse 5′-CCGTGG TCAGCATCTTGTTA-3′; RX forward 5′-GAATCTCGAAATCTCAGCCC-3′, reverse 5′-CTTCACTAATTTGCTCAGGAC-3′; SIX6 forward 5′-ATTTGGGACGGCGAACAG AAGACA-3′, reverse 5′-ATCCTGGATGGGCAACTCAGA TGT-3′; GAPDH forward 5′-ACCACAGTCCATGCCATCAC-3′, reverse 5′-TCCACCACCCTGTTGCTGTA-3′. Flow cytometry NR domains collected on D22 from two biological replicates were dissociated into single cells with trypsin, fixed in 1% PFA for 15 min, washed with PBS containing 0.04% triton-X-100 and 2% donkey serum, and then incubated for 1 h at room temperature in primary antibodies at a concentration of 1 μg of antibody per one million cells in PBS with 0.25% triton-X-100 and 2% donkey serum. Cells were then incubated with species-specific Alexa Fluor-488-conjugated secondary antibodies for 30 min, washed and analysed using a BD Accuri C6 Flow Cytometer (BD Pharmingen). In all experiments, nonspecific, species-appropriate isotype antibodies were used as controls. Data analysis was performed using BD Accuri C6 software. Ultrastructural analysis hiPSC-derived RCs were fixed in a cold, phosphate-buffered, 2.5% glutaraldehyde/2% PFA mixture, post fixed in 1% osmium tetroxide, dehydrated and embedded in Epon 812. Semi-thin sections were cut for orientation and ultra-thin sections (68 nm thickness) were cut and stained with uranyl acetate and lead citrate, and examined using a transmission electron microscope (Hitachi H7600). For quantification of developing outer-segment disc stacks, areas showing the apical side of the ONL were imaged at low magnification (× 1,000) and the length of the ONL was measured. Developing outer-segment discs stacks within these areas were identified at higher magnification (× 20,000). Four serial ultra-thin sections from a W27 CB-iPSC6.2-derived RC were analysed. Results are expressed as the average number of developing outer-segment discs stacks per 150 μm of ONL length. Live-cell imaging hiPSC-derived RCs were placed in a 1-mm-gap electroporation cuvette with a plasmid solution (2.3 μg μl −1 of pCIG plasmid expressing nuclear green fluorescent protein [68] in PBS) and four square pulses of 15 V, 50-ms duration and 950-ms interval were delivered using an ECM 830 electroporation apparatus (BTX, Holliston, MA, USA). Immediately after electroporation, RCs were returned to the cell-culture incubator for 36 h, at the end of which time-lapse microscopy imaging was performed at 2-h intervals for 48 h using an LSM 710 confocal laser scanning system (Zeiss) equipped with temperature and CO 2 control. Electrical recordings from photoreceptors in RCs In room light, CB-iPSC6.2-derived RCs (age W25–W27) were embedded in low-melting agarose gel and sliced into 100-μm-thick slices with a vibratome (Leica VT1000S). Next, in darkness, the eyecup slices were transferred to RC culture medium containing 100-μM 9- cis -retinal (a commercially available analogue of 11- cis -retinal) and incubated for 1 h in a light proof, 95% O 2 /5% CO 2 cell-culture incubator at 37 °C. Afterwards, the RC slices, still under light-proof conditions, were transferred and mounted laterally in the recording chamber. All procedures afterwards were performed in infrared or dim-red light. Perforated-patch recordings were performed at 35–37 °C on a Zeiss upright microscope equipped with infrared differential interference contrast (DIC) optics and imaging. The bath solution (Ames medium equilibrated with 95% O 2 /5% CO 2 ) was temperature controlled and ran at ~5 ml min −1 through the 1-ml experimental chamber. All recordings were in the voltage-clamp mode with V hold at −50 mV, low-pass filtered at 20 Hz (8-pole Bessel) and sampled at 500 Hz. The pipette solution contained (in mM): 110 KCl, 13 NaCl, 2 MgCl 2 , 1 CaCl 2 , 10 EGTA, 10 HEPES, 0.125 Amphotericin B, pH 7.2, titrated with KOH. The cells situated at the outer 1–4 layers of cells in the RC slice were chosen for recording because rod opsin-positive photoreceptors were concentrated in this region. The recorded photoreceptor was stimulated with diffuse white flashes (40-ms duration) from a mercury arc lamp, attenuated with neutral density filters, with intensity calibrated with a radiometer. Longitudinal analysis of hiPSC differentiation Formation of NR domains Aggregates seeded on D7 appeared as colonies under adherent culture conditions. Most colonies had clear boundaries before D20. The percentage of NR domains was evaluated by counting the number of VSX2-positive colonies among DAPI-positive colonies on D12, D16 and D20. Colonies containing >5 VSX2-positive colonies were considered NR domains. Results represent the average of three independent experiments, ~100 colonies per time point per cell line, per experiment. To trace the morphological progression of NR and RPE domains, plated aggregates were individually outlined using a microscope objective marker (Nikon) and imaged every other day from D17 to D25 under an inverted microscope (Nikon). Growth of RCs in long-term culture RCs were imaged every 15 days from D45 until D90 under inverted microscope with × 4 magnification. The length of the longest axis of RCs was measured using ImageJ. Results represent the average of 15–20 RCs per time point. Birthdating of retinal cell types To approximate the time of generation of the major retinal neuronal cell types, a minimum of five RCs were collected each week from W5 to W13, then every other week until W17, and once a month thereafter. Cell-type-specific markers were used for immunohistochemical identification as described above. Evaluation of RA effect on rod opsin expression RCs from the same culture batch were randomly assigned to the different treatment conditions. Initial analysis was carried out in CB-iPSC6.2-derived RCs by a semi-quantitative approach. Five RCs (three serial sections each) per treatment per time window were processed for immunohistochemical detection of rod opsin. Photoreceptor cells were considered ‘positive’ when rod opsin expression was clearly seen in the cell body (that is, cell membrane and/or cytoplasma). Results were expressed as: (−) no positive cells within RCs; (+) dispersed positive cells within RCs; (+++) patches of numerous positive cells within RCs. To compare the efficiency of generating rod-opsin-positive photoreceptor cells among the three hiPSC lines used in this study, W21 hiPSC-derived RCs subjected to W10–W14 RA treatment (8 to 22 RCs per cell line) were processed for immunohistochemical staining and analysed as described above. Results were expressed as the percentage of RCs showing positive rod opsin photoreceptors. How to cite this article: Zhong, X. et al . Generation of three-dimensional retinal tissue with functional photoreceptors from human iPSCs. Nat. Commun. 5:4047 doi: 10.1038/ncomms5047 (2014).